Palladium-catalyzed Suzuki-Miyaura coupling of thioureas or thioamides Cross-coupling reactions involving metal carbene intermediates play an increasingly important role in C–C bond formation. Expanding the carbene precursors to a broader range of starting materials and more diverse products is an ongoing challenge in synthetic organic chemistry. Herein, we report a Suzuki-Miyaura coupling reaction of in situ-generated Pd–carbene complexes via desulfurization of thioureas or thioamides. This strategy enables the preparation of a broad array of substituted amidinium salts and unsymmetrical diaryl ketones. The reaction is readily scalable, compatible with bromo groups on aromatic rings, tolerant to moisture and air and has a broad substrate scope. Furthermore, a single crystal structure of Pd-diaminocarbene complex is obtained and proven to be the key intermediate in both catalytic and stoichiometric reactions. Preliminary mechanistic studies demonstrate the dual role of the silver salt as a desulfurating reagent assisting the elimination of sulfur and as oxidant facilitating the Pd II /Pd 0 /Pd II catalytic cycle. In the past decade, the transition-metal-catalyzed carbene coupling reactions have emerged as one of the most powerful and reliable methods for carbon–carbon bond construction [1] , [2] , [3] , [4] , [5] , [6] , [7] , [8] , [9] , [10] , [11] , [12] , [13] , [14] , [15] . In most of these coupling reactions, diazo compounds were frequently employed to serve as very useful precursors for metal carbene generation, and many elegant transformations have been developed with diazo compounds, as a consequence, more and more chemists have been attracted to devote to this field [10] , [11] , [12] , [13] . In spite of the great advance and importance of diazo compounds in carbene coupling reactions, the discovery and development of carbene synthons which possess versatile reactivity and are stable, as well as convenient to prepare is still highly challenging [14] , [15] . In 2007, Barluenga et al. reported the first palladium-catalyzed carbene cross-coupling with tosylhydrazones (the precursors for in situ generated diazo compounds) [2] . Subsequently, they demonstrated a powerful reductive coupling of tosylhydrazones with boronic acids in the absence of a metal catalyst [3] . In addition, the allenyl ketones [5] , ene-yne-ketones [6] , alkynes [7] , cyclopropenes [8] along with chromium(0) Fischer carbene complexes [9] , have been proven as effective metal carbene precursors in cross-couplings by Wang and co-workers, which have prominently enriched the toolboxes of synthetic chemists (Fig. 1a ). In 1993, Kuhn and co-workers [16] , [17] , [18] reported an efficient method for the synthesis of metal N -heterocyclic carbene (NHC) complexes: it involves the synthesis of NHC complexes via desulfurization of imidazole-derived thioureas in the first step, and subsequent coordination to corresponding metal salts. Such desulfurization of thioureas needs stoichiometric amounts of potassium or sodium as desulfurating reagents via the removal of K 2 S or Na 2 S. However, the stoichiometric alkali metals, harsh reaction conditions and limited scope of acyclic thioureas restricted their application in organic synthesis, especially in metal-catalyzed organic reactions. In addition, Yang et al. have recently demonstrated that thioureas can serve as ligands to a variety of different transition-metal-catalyzed reactions, because of the strong coordinative and adsorptive properties of the sulfur atom, and they have also found their application in the total synthesis of natural products [19] . In 2005, Fürstner et al. reported the elegant synthesis of metal-diaminocarbene complexes C (from thioureas) or metal-monoaminocarbene complexes C′ (from thioamides) by oxidative addition of electron-rich metal centers (e.g., Pd 0 , Ni 0 ) into the Vilsmeier-type salts B , which were prepared from thioamide derivatives A and oxalyl chloride (Fig. 1b ) [20] . For the reactivity of metal-aminocarbene complexes, Grushin, Yates and Cavell demonstrated that the alkyl/aryl/acyl-carbene reductive elimination from imidazole-derived Pd II heterocylic carbene complexes, as the side reaction in metal-NHC system, could lead to catalyst deactivation along with undesired carbon–carbon bond formation [21] , [22] , indicating that the reaction of metal-aminocarbene and its ligand prefer carbene reductive elimination to carbene migratory insertion. Fig. 1: Direct desulfurization for the generation of carbenes. a Transition-metal-catalyzed carbene coupling reactions by carbene migratory insertion. M = metal. b Our concept for the catalytical generation of metal-aminocarbene from thioamide derivatives A and its crossing coupling reactions. c Hypothesis of mechanism for desulfurative Suzuki–Miyaura coupling reaction based on Pd 0 /Pd II /Pd 0 catalytic cycle by carbene reductive elimination. X − = anion; L = Ligand. Full size image In continuation of our work on the reactivity of the thioamide-derived substrates [23] , [24] and inspired by Kuhn’s NHCs synthesis, we are intrigued by the possibility of the thioamide derivatives (thioureas can be regarded as two parts of thioamide) as metal carbene precursors. The use of thioamide derivatives A for the catalytical generation of metal-aminocarbenes through the elimination of sulfide is particularly appealing and is expected to offer great opportunities, especially when it leads to unconventional reaction mechanism and unique retrosynthetic relationships (Fig. 1b ). To elaborate the feasibility of our plan, we propose a plausible mechanism depicted in Fig. 1c , which involves Pd 0 /Pd II /Pd 0 catalytic cycle. Generally, the reversible intermediate D can be easily generated from thioamide A as a result of the coordination of thiophile (or thiophilic auxiliary) [25] , [26] , [27] , [28] , [29] , which leads to oxidative addition of the C–S bond [30] , [31] , [32] , [33] , [34] , [35] in the presence of active L n Pd 0 , affording the formal sulfur-containing metal-aminocarbene intermediate in equilibrium between the cationic form E and the neutral form F or F′ (not shown in Fig. 1c ) [20] . The development of a catalytic version of this type of reactions from thioamide derivatives remains a formidable challenge, probably due to the high-energy barrier in desulfurization process, the poor compatibility of desulfurating reagents with substrates and the difficulty in finding a suitable condition and appropriate metal which can not only capture the in situ -generated carbene species but also accomplish the catalytic crossing-coupling cycle, meanwhile, the metal catalyst can’t be poisoned by sulfur species. Given the commercial availability, stability, and nontoxicity of organoboron reagents, transition-metal catalyzed Suzuki−Miyaura coupling (SMC) will be an ideal choice for achieving the aforementioned catalytic cycle [36] , [37] , [38] , [39] , [40] , [41] , [42] , [43] , [44] . Thus, the coupling of the Pd-aminocarbene complex with organoboron II compound can in principle produce the iminium salt intermediate G via reductive elimination, which will set the stage for the preparation of a broad array of substituted amidinium salts (from thioureas) and unsymmetric ketones (from thioamides). Remarkably, the amidinium salts are prevalent in many functional molecules or materials and bioactive molecules [45] , [46] , [47] , [48] (Fig. 2 ), such as amidinium salt I (a hydrogen-bond donor to activate electron-deficient quinones and a catalyst in a quinone-mediated model synthetic transformation) [45] , amidinium salt II (antistatic agent) [46] , III (alkaline-stable benzimidazolium in high-performance hydroxide conducting membranes) [47] and amidinium salt IV (antifungal agent) [48] . Moreover, amidinium salts are a well-known subclass of ionic liquids (ILs) [49] , [50] . Fig. 2 Selected compounds containing amidinium salt unit. The significance of amidinium salts I – IV . Full size image Herein, we now report a successful example of the use of an in situ- generated Pd−carbene complex through desulfurization of thioureas or thioamides to accomplish Suzuki−Miyaura coupling reaction to afford a broad array of substituted amidinium salts or valuable diaryl ketones. 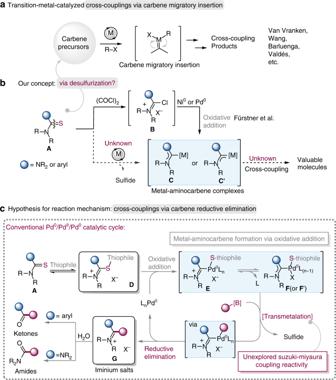Fig. 1: Direct desulfurization for the generation of carbenes. aTransition-metal-catalyzed carbene coupling reactions by carbene migratory insertion. M = metal.bOur concept for the catalytical generation of metal-aminocarbene from thioamide derivativesAand its crossing coupling reactions.cHypothesis of mechanism for desulfurative Suzuki–Miyaura coupling reaction based on Pd0/PdII/Pd0catalytic cycle by carbene reductive elimination. X−= anion; L = Ligand. Synthetic methodology development Firstly, after detecting the formation of amide phenyl(piperidin-1-yl)methanone ( 3 ) in 15% yield (Table 1 , entry 2) by using di(piperidin-1-yl)methanethione ( 1a ) and phenyl boronic acid ( 2a ) as the model substrates, we next investigated the effect of Pd catalysts and found that common Pd(PPh 3 ) 2 Cl 2 was the best choice (Table 1 , entries 1–5). According to the related reports, the desulfurization of thioamide derivatives were efficiently performed with Ag 2 CO 3 [25] , CuSO 4 •5H 2 O [26] , CoCl 2 •6H 2 O [27] , and PhI(OAc) 2 [28] by the formation of Ag 2 S, CuS, CoS and elemental sulfur respectively. Screening of common desulfurating reagents showed that Ag 2 CO 3 exhibited best activity (Table 1 , entries 5–9). To facilitate transmetallation of phenyl boronic acid, a series of additional bases was also studied and Na 2 CO 3 was the optimal one (entries 11–13). The amount of Pd catalyst as well as the silver salt loading and base usage highly affected the efficiency of this transformation. When submitting 1a and 2a along with 10 mol% of Pd(PPh 3 ) 2 Cl 2 in trifluoroethanol (TFE, without dehydration) under air atmosphere with 1.5 equivalents of Ag 2 CO 3 , a 93% yield of the amide phenyl(piperidin-1-yl)methanone ( 3 ) could be obtained (Table 1 , entry 16). Silver salt was essential for the success of this reaction (Table 1 , entry 17). Based on our proposed mechanism, the hydrolysis of intermediate G can provide amide using thiourea as the substrate (Fig. 1c ). To capture the intermediate G , we tried to add two equivalents of HOTf into the reaction system without workup. 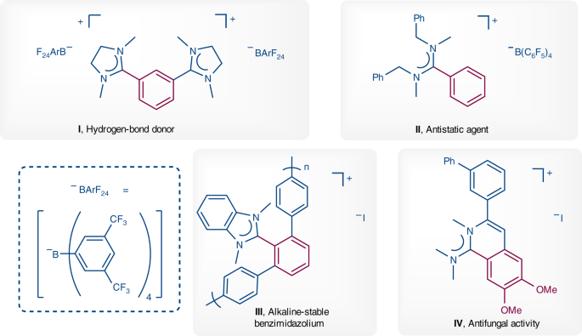Fig. 2 Selected compounds containing amidinium salt unit. The significance of amidinium saltsI–IV. Fortunately, we found the amidinium salt 4 with OTf anion was obtained in 98% yield (Table 1 , entry 19) and its structure has been unambiguously confirmed by X-ray crystallographic analysis (Table 2 , CCDC 1895265). Table 1 Optimization of reaction conditions. Full size table Table 2 Substrate scopes with respect to the construction of amidinium salts a . Full size table Substrate scope with respect to amidinium salts With the optimized reaction conditions (Table 1 , entry 19) in hand, we investigated the substrate scope of the construction of amidinium salts first (Table 2 ). In general, boronic acids bearing both electron-donating (e.g., –Me, – i Pr, –OEt, –Ph) and electron-withdrawing groups (e.g., –F, –Cl, –CN) on the aromatic rings could react smoothly to produce amidinium salts in good yields ( 4 – 12 , 18 – 19 ). It is noteworthy, yet very unusual in palladium chemistry, that bromo-substituted boronic acids were tolerated well under our conditions ( 13 and 20 ), and this provides an extremely important choice for cross-coupling reactions and makes the further structural elaboration feasible. Significantly, boronic acids bearing versatile functional groups, such as –OH, –CHO, –Ac, and –COOEt are competent reaction partners as well ( 8 , 15 – 17 ). Polyphenylene species, like naphthalene and 9,9-dimethyl-9 H -fluorene were also amenable motifs ( 21 – 22 ). Heteroaromatic substrates, such as unprotected indole and dibenzo[b,d]thiophene were successfully converted to the corresponding products in 73–76% ( 23 and 24 ). Next, we investigated the effect of substituents on thioureas. Good results were obtained with di(pyrrolidin-1-yl)methanethione and 1,1,3,3-tetramethyl-thiourea ( 25 and 26 ). Expanding the scope to the cyclic thioureas was also effective, affording five-, six-, and seven-membered amidinium salts in 86%, 76%, and 90% yield, respectively ( 27 – 29 ). Notably, ortho substituted boronic acids also exhibited acceptable reactivity, although corresponding amidinium salts were obtained in lower yields ( 30 and 31 ). Importantly, unsymmetric thioureas were also good candidates in this method, featuring the positive ion delocalization in N–C–N triple atom ( 32 and 33 ). Considering the importance of carbazole moiety [51] (organic light emitting diodes, OLEDs), Amoxapine [52] (antidepressant) and Cytisine [53] within optoelectronic materials, drugs, or natural products, we synthesized the structurally complex amidinium salts in satisfactory yield ( 34 – 36 ) using corresponding substrates bearing thiourea units. Moreover, estrone-derived arylboronic acid pinacol ester could also smoothly convert to amidinium salt 37 in 92% yield, indicating that our protocol enables a practical late-stage modification in medicinal chemistry. Substrate scope with respect to diaryl ketones The existence of Pd II -monoaminocarbene complexes [20] and the success of above reactions prompted us to expand this catalytic system to more general thioamide-containing substrates. Thioamides can be easily obtained by different functional group transformation, meanwhile, they also serve as versatile building blocks to provide valuable compounds [54] . Conventionally, Lawesson’s reagent and its analogues are employed to the synthesis of thioamides, starting from aryl amides, aryl carboxylic acids, and nitriles [55] . Willgerodt–Kindler reaction is another alternative means to access thioamides, starting from different types of starting materials such as aryl aldehydes, aryl alkyl ketones, aryl amides, and aryl acetic acids in one step [56] , [57] . It means that these common compounds can conveniently be used to prepare diaryl ketones in two steps with our method, which can enlarge the accessible chemical space. Although different strategies have been developed, alternative syntheses of diaryl ketones, which can commendably deal with the problem of chemoselectivity and poor functional group compatibility [58] , [59] , are still highly desirable and a pursued goal in the synthetic field [39] , [41] . 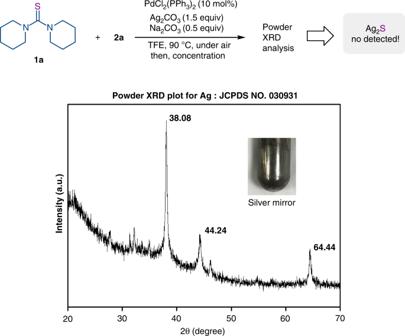Fig. 3 Powder XRD analysis of the reaction mixture. (inset) The photo of the silver mirror. Our primary studies on the reaction of thioamide with phenyl boronic acid ( 2a ) also gave positive results through employing the Cu(OAc) 2 •H 2 O as additive instead of Ag 2 CO 3 (Table 3 ). Using 7.5 mol% PdCl 2 (PPh 3 ) 2 , thioamides smoothly reacted with aryl boronic acids to afford both symmetric and unsymmetric diaryl ketones in medium to excellent yields (Table 3 , 38 – 89 ). This transformation exhibited an excellent functional group tolerance. In addition to alkyl groups, halo, vinyl, ketone, ester, cyano, nitro, hydroxyl groups, complex structure (adapalene), as well as heterocycles such as indole, thiophene, pyridine and quinolone were all tolerated well. Again, bromine substituted substrates were not impeded by our catalytic protocol, thus indicating that the activation of thiourea or thioamide was prior to the oxidative addition of aryl bromide by Pd catalysis. Next, a potent antiproliferative agent [60] 88 was readily obtained in 63% yield from the corresponding thioamide and indolyboronic acid under the standard coupling conditions. Fenofibrate, a cholesterol-modulating drug [61] , could be obtained in 90% yield under similar operation (Table 3 , 89 ). Table 3 Substrate scope of simple and efficient synthesis of diaryl ketones. a Full size table Mechanistic investigation On the basis of the aforementioned reaction mechanism (Fig. 1c ) and relevant reports, this coupling would in principle produce one molecule of Ag 2 S to finish the transmetalation with organoboron compound [25] , [26] , [27] , [28] , suggesting that the silver should not change in valence state. Remarkably, the black colored precipitate, collected after the reaction through direct concentration in vacuo, was characterized by the powder XRD analysis (X-ray diffraction analysis); notably, no Ag 2 S (JCPDS 14–72) was detected. As can be seen from Fig. 3 , it is a clear indication for the existence of elemental silver in the powder X-ray analysis picture, which well matched the standard XRD pattern of elemental silver (JCPDS No.030931). Moreover, we also observed a silver mirror during the reaction, indicating that the Ag salt would serve as an oxidant to furnish the catalytic cycle. Fig. 3 Powder XRD analysis of the reaction mixture. (inset) The photo of the silver mirror. Full size image To demonstrate the detailed reaction process, several control experiments were performed. When urea 90 was exposed to the standard conditions, no reaction occurred, suggesting the necessity of the unique structure of thiourea for the success of the transformation (Fig. 4a , eq 1). In order to identify the fate of sulfur element and to intercept the possible Pd intermediates, the thiourea 1a was mixed with a stoichiometric amount of PdCl 2 (PPh 3 ) 2 and 1.5 equiv of Ag 2 CO 3 at 90 °C for 4 h. Surprisingly, only in the presence of Ag 2 CO 3 , triphenylphosphine sulfide 91 was isolated in 51% yield (PhSPh was also detected under the catalytic reaction, please see the Supplementary Fig. 4 ). We speculated that the elemental sulfur might be generated during the reaction and then was captured by the triphenylphosphine (released from the Pd catalysis) (Fig. 4b , eq 2 left). Indeed, the PPh 3 was readily sulfurized in TFE to triphenylphosphine sulfide 91 in 95% yield (Fig. 4b , eq 2 right). Fig. 4: Insights into the reaction mechanism. a Transformation of urea 90 . b Mechanistic investigation. c The proposed mechanism. Full size image After filtration of inorganic solids and addition of ether solvent, yellow crystal 94 was precipitated and separated, and the unique carbene structure was confirmed by X-ray crystallography (Fig. 4b ). All these operations were conducted under air atmosphere. 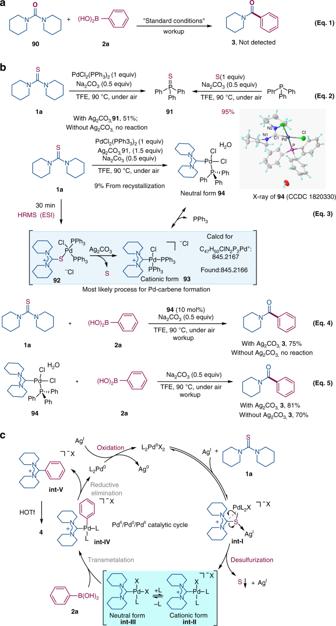Fig. 4: Insights into the reaction mechanism. aTransformation of urea90.bMechanistic investigation.cThe proposed mechanism. 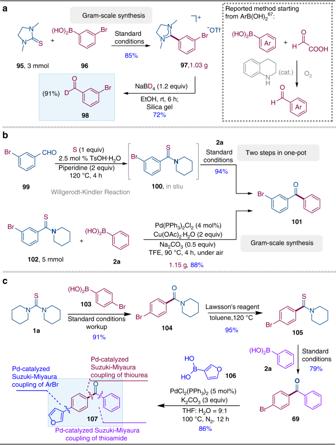Fig. 5: Synthetic applications. aConcise synthesis of deuterated aldehyde98.bOne-pot synthesis of ketone101via Willgerodt-Kindler reaction and gram-scale synthesis of ketone101.cOrthogonal coupling for three different C–C bonds formation. The square structure of this complex indicates it is a cis -configured Pd II species (CCDC 1820330). The bond lengths of Pd-C1 (2.004 Å), C1-N1 (1.339 Å) and C1-N2 (1.325 Å), as well as the N–C-N angle (122.8°) are consistent with those known similar acyclic diaminocarbene-Pd complexes [20] , meanwhile, the two C–N bond lengths (1.339 Å and 1.325 Å) are typical C=N bond length, it sufficiently suggested the phenomenon of electron delocalization in N–C–N triple atom system (Fig. 4b , eq 3). Moreover, the HRMS (high resolution mass spectrometry) analysis of the mixture of the standard reaction for 30 min showed the distinctive Pd peak at m/z = 845.2166, which matched the cationic form intermediate 93 (calcd mass: 845.2167). According to the control experiment (Table 1 , entry 17), the Ag salt would play dual roles in this transformation: it acts as a thiophilic auxiliary for desulfurization to form metal-aminocarbene complex, at the same time, it also serves as an oxidant to oxidize Pd 0 to Pd II to furnish the catalytic cycle. Next, complex 94 catalyzed the Suzuki−Miyaura reaction under the standard conditions in the presence of Ag 2 CO 3 delivering benzamide 3 in high yield, suggesting the plausible intermediacy of it in the catalytic cycle (Fig. 4b , eq 4). Not surprisingly, in the absence of Ag 2 CO 3 , there was no product 3 detected. The reaction between stoichiometric amount of complex 94 and arylboronic acid 2a was performed subsequently under the standard conditions (Fig. 4b , eq 5), rendering 3 in 81% yield (with Ag 2 CO 3 ) or in 70% yield (without Ag 2 CO 3 ), which further confirmed the possibility that complex 94 is the key intermediate in our transformation. Moreover, to get more insight into the reaction mechanism, the dependence of the initial rate on the concentrations of thiourea, PhB(OH) 2 ( 2a ), PdCl 2 (PPh 3 ) 2 and Ag 2 CO 3 were examined respectively (see Supplementary Figs. 6 – 13 ). Zero-order relationships of the initial rate with the concentration of thiourea and PhB(OH) 2 were observed. A first-order dependence of the initial rate on the amount of the palladium catalyst was established. For Ag 2 CO 3 , there was an induction phase observed in initial rate–concentration plots. After the induction phase, the reaction is clearly first order in Ag 2 CO 3 . Proposed mechanism On the basis of the aforementioned results, a plausible mechanism, based on silver-facilitated Pd II /Pd 0 /Pd II catalytic cycle (for the possibility of heterogeneous Pd catalysis, see Supplementary Fig. 5 ), is depicted in Fig. 4 . First, the reversible intermediate int-I is formed via coordination or complexation [62] , [63] of L 2 Pd II X 2 with substrate ( 1a ) in the presence of a silver salt [25] , which leads to Ag I -facilitated desulfurization to produce the Pd II -diaminocarbene intermediate along with the expulsion of sulfur and Ag I salt (or their complex). We consider that sulfur-extrusion reaction is similar to the decarbonylation [64] , desulfitation and decarboxylation [65] , [66] . Next, The intermediate is in equilibrium between the cationic form int-II and the neutral form int-III , which involves the displacement of ligand on intermediate int-II by the nucleophilic X − anion, yielding the neutral cis -form int-III [22] . With the presence of phenyl boronic acid ( 2a) , the Pd II -species int-IV is generated via the transmetalation. According to the related studies [21] , [22] from Yates and Cavell, the C–C bond formation of Pd II -species int-IV could occur with a low activation barrier, proceeding via a concerted reductive elimination of the aryl and carbene moiety. Thus, the desired amidinium salt int-V is released through reductive elimination on Pd II center to Pd 0 species; once again, the Ag I salt produced by desulfurization step would also serve as an oxidant to oxidize Pd 0 to Pd II to furnish the catalytic cycle with the Ag 0 (elemental silver) as by-product, which is consistent with the experimental results (Fig. 4c ). Further applications With the development of the Pd-catalyzed Suzuki–Miyaura coupling of thioureas and thioamides, we decided to pursue their applications (Fig. 5 ). Firstly, A gram-scale version of the reaction using cyclic thiourea 95 (3 mmol) and 3-bromophenylboronic acid 96 was performed, and the desired amidinium salt 97 was obtained in 85% yield on 1.03 g scale (Fig. 5a ). Next, deuterated aromatic aldehyde 98 (91% deuterated ratio) was obtained in 72% via the reduction of amidinium salt 97 using NaBD 4 and subsequent hydrolysis. Very recently, the synthesis of aromatic aldehydes from arylboronic acids was firstly reported by Mariano and co-workes [67] via organocatalytic formylation reactions of boronic acids with glyoxylic acid. To the best of our knowledge, the synthesis of deuterated aromatic aldehydes from arylboronic acids, even if it takes two steps, has never been reported before, which leads to unique retrosynthetic relationship. To further demonstrate the practicability of our method, we have also developed a one-pot protocol starting directly from aldehydes. For example, 3-bromobenzaldehyde ( 99 ) could be converted to the corresponding thioamide via Willgerodt-Kindler reaction in one step [68] , no further purification is required, 2a , Pd catalyst, Cu salt, Na 2 CO 3 and TFE were added to the same reaction flask, and the corresponding cross-coupling product 101 was obtained in 94% yield in two steps after stirring the mixture at 90 o C for 4 h under air (Fig. 5b ). A gram-scale version of the reaction using brominated substrates 102 and 2a was also carried out, and the desired ketone 101 was obtained in 88% yield on 1.15 g scale using only 4 mol % PdCl 2 (PPh 3 ) 2 (Fig. 5b ). Moreover, a sequential Pd-catalyzed Suzuki–Miyaura couplings starting from thiourea 1a was carried out in Fig. 5c . Thiourea 1a was first coupled with para -bromo-phenylboronic acid 103 , and amide 104 was obtained in 91% yield, leaving bromo group untouched. Lawsson’s reagent readily converted amide 104 into thioamide 105 , which further underwent a Pd-catalyzed Suzuki–Miyaura coupling with phenylboronic acid 2a , rendering ketone 69 in 79% yield, once again, bromo group on aromatic ring was remained intact. A third Suzuki–Miyaura coupling between 69 and 3-furanylboronic acid 106 was performed, furnishing a ketone 107 in 86% yield. Therefore the combination of three Suzuki–Miyaura reactions provides the free design of ketones with three different C–C bonds formation from the resource of boronic acids, while simple thiourea species donates a carbonyl bridge. Fig. 5: Synthetic applications. a Concise synthesis of deuterated aldehyde 98 . b One-pot synthesis of ketone 101 via Willgerodt-Kindler reaction and gram-scale synthesis of ketone 101 . c Orthogonal coupling for three different C–C bonds formation. Full size image In summary, we have reported a Suzuki–Miyaura coupling reaction of thioureas or thioamides to afford a broad array of substituted amidinium salts or valuable diaryl ketones. Inspired by the stoichiometric carbene-generating methods, we successfully realize the direct generation of metal–carbene complex in a catalytic manner. Single crystal structure of Pd-diaminocarbene complex is obtained and proven to be the key intermediate by both catalytic and stoichiometric reactions. Meanwhile, HRMS analysis further supports our hypothetical intermediates for reaction mechanism. Preliminary mechanistic studies demonstrate the dual roles of silver salt: (i) a desulfurating reagent that assist the elimination of sulfur; (ii) an oxidant that facilitate the Pd II /Pd 0 /Pd II catalytic cycle. Further studies on expansion of this reaction to other substrates to achieve anothercoupling reactions as well as the development of this carbene chemistry are underway in our laboratory. General procedure for the synthesis of amidinium salts Thiourea (0.2 mmol, 1.0 equiv), aryl boronic acid (0.4 mmol, 2.0 equiv), PdCl 2 (PPh 3 ) 2 (14.0 mg, 0.02 mmol, 10 mol %), Ag 2 CO 3 (82.7 mg, 0.3 mmol, 1.5 equiv), Na 2 CO 3 (10.6 mg, 0.1 mmol, 0.5 equiv), and TFE (1.5 mL), were placed in a 50 mL Schlenk sealed tube (with a Teflon cap) equipped with a magnetic stir bar. The reaction was stirred at 90 o C for 4 h under air. Subsequently, the reaction mixture was cooled to room temperature and HOTf (60 mg, 0.4 mmol, 2 equiv) was added. The crude reaction mixture was concentrated in vacuo, and the residue was purified by flash chromatography on silica gel to provide the desired amidinium salts using CH 2 Cl 2 /MeOH as the eluent. General procedure for the synthesis of amide 3 Thiourea (0.2 mmol, 1.0 equiv), aryl boronic acid (0.4 mmol, 2.0 equiv), PdCl 2 (PPh 3 ) 2 (14.0 mg, 0.02 mmol, 10 mol %), Ag 2 CO 3 (82.7 mg, 0.3 mmol, 1.5 equiv), Na 2 CO 3 (10.6 mg, 0.1 mmol, 0.5 equiv), and TFE (1.5 mL), were placed in a 50 mL Schlenk sealed tube (with a Teflon cap) equipped with a magnetic stir bar. The reaction was stirred at 90 o C for 4 h under air. Subsequently, the reaction mixture was cooled to room temperature and 1 M HCl (10 mL) was added. The mixture was then extracted with EtOAc. The organic layer was concentrated in vacuo, and the residue was purified by flash chromatography on silica gel to afford the amide 3 using petroleum ether/EtOAc as the eluent. General procedure for the synthesis of diaryl ketones Thioamide (0.2 mmol, 1.0 equiv), aryl boronic acid (0.4 mmol, 2.0 equiv), PdCl 2 (PPh 3 ) 2 (10.5 mg, 0.015 mmol, 7.5 mol %), Cu(OAc) 2 ·H 2 O (79.9 mg, 0.4 mmol, 2 equiv), Na 2 CO 3 (10.6 mg, 0.1 mmol, 0.5 equiv), and TFE (1.5 mL), were placed in a 50 mL Schlenk sealed tube (with a Teflon cap) equipped with a magnetic stir bar. The reaction was stirred at 90 o C for 4 h under air. Finally, the reaction mixture was cooled to room temperature and the crude reaction mixture was concentrated in vacuo. The remaining residue was purified by flash chromatography on silica gel to afford the diaryl ketones using petroleum ether/EtOAc as the eluent.